Lithium–sulphur batteries with a microporous carbon paper as a bifunctional interlayer The limitations in the cathode capacity compared with that of the anode have been an impediment to advance the lithium-ion battery technology. The lithium–sulphur system is appealing in this regard, as sulphur exhibits an order of magnitude higher capacity than the currently used cathodes. However, low active material utilization and poor cycle life hinder the practicality of lithium–sulphur batteries. Here we report a simple adjustment to the traditional lithium–sulphur battery configuration to achieve high capacity with a long cycle life and rapid charge rate. With a bifunctional microporous carbon paper between the cathode and separator, we observe a significant improvement not only in the active material utilization but also in capacity retention, without involving complex synthesis or surface modification. The insertion of a microporous carbon interlayer decreases the internal charge transfer resistance and localizes the soluble polysulphide species, facilitating a commercially feasible means of fabricating the lithium–sulphur batteries. Entering a new era of green energy, several criteria such as cost, cycle life, safety, efficiency, energy and power need to be considered in developing electrical energy-storage systems for transportation and grid storage [1] . Lithium–sulphur (Li–S) batteries are one of the prospective candidates in this regard, as sulphur offers a high theoretical capacity of 1,675 mA h g −1 at a safer operating voltage range of ~2.1 V and lower cost compared with the currently used oxide and phosphate cathodes. With this perspective, there is increasing interest in recent years in the Li–S battery research. Development of a high capacity (>800 mA h g −1 ) Li–S system with a long, acceptable cycle life will give this system a greater opportunity to be commercialized in the near future [2] , [3] , [4] , [5] . The early-stage research in Li–S batteries was initiated three decades ago [6] , [7] , but the spotlight did not return to this battery system until there was a renewed interest in electric vehicles in recent years. The major impediments to the development of Li–S batteries are low active material utilization, poor cycle life and low charge efficiency [8] . The poor utilization of active material results from the insulating sulphur, which hinders the electron transfer during electrochemical reactions. Also, sulphur molecules form easily dissolved polysulphide intermediates with lithium (Li 2 S x , 2<x≤8) in the electrolyte, resulting in severe capacity fade [9] , [10] . The soluble polysulphides shuttling between the anode and cathode lead to low Coulombic efficiency [11] , [12] . Thus, improving the conductivity of the sulphur cathode and maintaining/re-utilizing soluble polysulphides within the cathode structure are critical to develop a viable Li–S system. Employing sulphur–carbon composites and applying conductive polymer surface modification are the main approaches in laboratories around the world to realize high capacity and improved cycle life [2] , [3] , [4] , [5] , [13] , [14] , [15] , [16] , [17] , [18] , [19] , [20] . Both approaches enhance the electrical conductivity of the cathode and suppress the loss of soluble polysulphide intermediates during cycling and thereby improve the active material utilization and cyclability. In addition, the issue of low Coulombic efficiency has been resolved by the addition of lithium nitrate to the electrolyte [5] , [21] . As discussed, the major stream of the Li–S battery research has focused on the modification ‘inside’ of the cathode and electrolyte, but the design ‘outside’ of the cathode, such as cell configuration, could be a new strategy for improving the performance of the Li–S batteries. On the basis of the fact that porous carbon has a key role, both as electron pathways and as traps for dissolved polysulphide species, we present here an insertion of an electrolyte-permeable microporous carbon paper (MCP) between the separator and cathode disk to improve the electrochemical performance of the Li–S cells. This design of cell configuration can effectively decrease the resistance of sulphur cathodes, resulting in an enhancement of active material utilization. In addition, the carbon interlayer with micropores used in this study facilitates the absorption of soluble polysulphides shuttling in the electrolyte and makes them available to be reutilized even during long cycles. This bifunctional carbon interlayer can be treated as a second current collector for accommodating the migrating active material from sulphur cathodes. This novel approach not only simplifies the battery processing without elaborate synthesis of composites and surface chemistry modification, but also improves the capacity and cycle life, thereby promoting the practicality of Li–S batteries. Cell configuration of the Li/MCP interlayer/S battery The battery configuration of a Li–S cell with a bifunctional microporous carbon interlayer is displayed in Fig. 1a . The conductive carbon interlayer has to be placed between the separator and cathode to capture the migrating polysulphides (Li 2 S x ) from the cathode during electrochemical reactions, but without contacting the Li anode. Here we employ pure sulphur powder as the active material to make conventional sulphur cathodes instead of using specialized composites or adopting any surface chemistry modification to demonstrate that the observed improvement in cyclability is only contributed by the carbon interlayer. 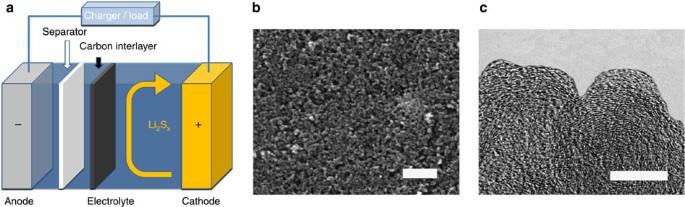Figure 1: Scheme and morphology of the MCP employed in the Li–S battery. (a) Schematic configuration of a Li–S cell with a bifunctional microporous carbon interlayer inserted between the sulphur cathode and the separator, (b) SEM image of the surface of the MCP and (c) transmission electron microscope image of the microporous carbon particles. The scale bars inbandcequal 500 nm and 10 nm, respectively. Figure 1b shows the scanning electron microscope (SEM) image of the MCP used in this study as the interlayer. It can be seen that the carbon particles in the film is nano-sized, which is able to provide subtle surface contact with the sulphur cathode to reduce the electrical resistance. In addition, the interlayer surface is highly porous, resulting in good electrolyte penetration during cycling. The particle size of the carbon nanoparticles in the MCP ranges between 20 and 40 nm ( Fig. 1c ), and no mesopores with a diameter >5 nm can be found in the carbon. Figure 1: Scheme and morphology of the MCP employed in the Li–S battery. ( a ) Schematic configuration of a Li–S cell with a bifunctional microporous carbon interlayer inserted between the sulphur cathode and the separator, ( b ) SEM image of the surface of the MCP and ( c ) transmission electron microscope image of the microporous carbon particles. The scale bars in b and c equal 500 nm and 10 nm, respectively. Full size image Pore-filling process of the MCP interlayer during cycling The nitrogen adsorption/desorption isotherms of MCP as the interlayer in Li–S batteries before and after cycling are displayed in Fig. 2a . It can be seen that both the microporous carbon powder and MCP exhibit mixed type I and type II isotherms, respectively, for low relative pressure ( P / P 0 ) and high P / P 0 [22] , [23] . The raw microporous carbon powder and MCP have certain nitrogen adsorption below the relative pressure of P / P 0 <0.1, indicating the existence of micropores [22] . The rise after P / P 0 >0.9 represents the integral porosity of MCP contributed by the interspaces between the carbon nanoparticles, offering abundant channels for liquid electrolyte. The amount of mesopores is limited because of the gentle adsorption slope at P / P 0 =0.1–0.9. The MCP as the interlayer after cycling shows almost zero adsorption at the micropore region, demonstrating that these micropores are filled during the discharge/charge of the Li–S cells. A depletion of the hysteresis loop is found in the cycled MCP, also indicating a portion of mesopores are filled. The total surface area of pristine MCP is as high as 695 m 2 g −1 (65% contributed by micropores), but that of the MCP after cycling is only 61 m 2 g −1 due to the filling of the pores in the interlayer. The total pore volume of MCP after 100 cycles is as low as 0.288 cm 3 g −1 (no micropore volume), which is much less than that of pristine MCP (1.194 cm 3 g −1 ; 0.215 cm 3 g −1 for micropore volume). 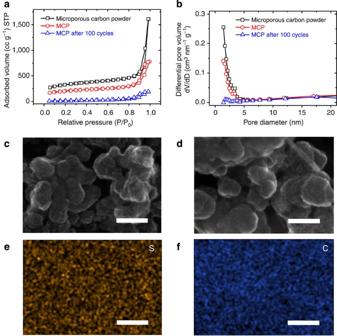Figure 2: Surface area, morphology and elemental analyses of the MCP. (a) Isotherms and (b) pore size distributions of the microporous carbon powder, MCP, and MCP as an interlayer in the Li–S cell at 1C rate after 100 cycles. SEM images of the MCP (c) before cycling and (d) after cycling. Elemental mapping of (e) sulphur and (f) carbon ind. The scale bars inc–fequal 50 nm. Figure 2b exhibits the pore size distributions of the MCP samples, where all specimens have no obvious pores with a diameter over 5 nm. These curves end at the pore diameter below 1.4 nm because of the limitation of the analyser. The microporous/small-mesoporous peak of the MCP almost vanishes after cycling, implying that the migrating active polysulphides might be captured and might fill these pores during the electrochemical cycling. Figure 2: Surface area, morphology and elemental analyses of the MCP. ( a ) Isotherms and ( b ) pore size distributions of the microporous carbon powder, MCP, and MCP as an interlayer in the Li–S cell at 1C rate after 100 cycles. SEM images of the MCP ( c ) before cycling and ( d ) after cycling. Elemental mapping of ( e ) sulphur and ( f ) carbon in d . The scale bars in c–f equal 50 nm. Full size image Surface morphology and elemental analysis of the MCP interlayer Figure 2c compare the SEM images of the MCP interlayer surface towards the cathode before and after cycling. Pristine MCP in Fig. 2c exhibits a morphology of glue-like particles composed of microporous carbon and binder. The MCP after 100 cycles still has spherical morphology with individual microporous carbon particles, showing that the dissolved active material is probably absorbed by the pores in the interlayer rather than forming large insulating S/Li 2 S-inactive layers. This feature is critical because irreversible capacity loss would occur if active material agglomerates and non-uniformly covers the cathode, which can block charge transfer reactions and ion transport in the cell [9] , [10] . The surface porosity of the MCP after cycling is still maintained, which guarantees the infiltration of electrolyte. Figure 2e display the elemental mapping results of the MCP interlayer after cycling. Sulphur signal is found all over the carbon interlayer and distributed homogenously, ensuring a superior re-utilization of the active material and reversibility. Moreover, it is noteworthy to mention that the carbon signal is also well distributed and strong in the interlayer, indicating that the conductive carbon is not severely covered by sulphur/sulphides and leading to good conductivity in the cathode region even for long cycles. Electrochemical performance of the Li–S batteries with the MCP interlayer To analyse the impact of the MCP as the carbon interlayer in Li–S batteries, impedance analysis was performed to compare the cells with and without the MCP interlayer before cycling ( Fig. 3a ). The impedance of Li–S batteries located in the high-frequency region is regarded as the charge transfer resistance of the cell [24] . The impedance semi-circle shrinks significantly by about 79% after the insertion of the MCP, demonstrating a dramatic decrease in the charge transfer resistance of the battery. Here, the MCP interlayer works as an upper current collector for the low-conductivity sulphur cathode, enhancing the active material utilization and thereby raising the specific capacity of the cell. 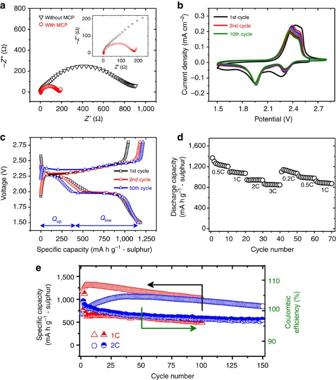Figure 3: Electrochemical measurements of Li–S batteries. (a) Electrochemical impedance spectroscopy plots of Li–S cells with and without MCP, (b) cyclic voltammogram scans, (c) discharge/charge profiles at various cycles, (d) rate capability up to 3C and (e) cycle life and Coulombic efficiency of the cell with MCP at 1C and 2C for long cycles. Figure 3b shows the cyclic voltammograms of the cell with the MCP for the first ten cycles. Two cathodic peaks at around 2.3 and 2.0 V, and the two overlapped anodic peaks at around 2.35 and 2.45 V are typical of Li–S cells with carbon-based cathodes [2] , [15] . The overpotential of the first cathodic peak disappears after the first cycle, possibly due to the rearrangement of the migrating active material to electrochemically favourable positions. The discharge/charge profiles in Fig. 3c , exhibiting two discharge plateaus and two closely spaced charge plateaus, are consistent with the cyclic voltammogram plots. The upper discharge plateau represents the transformation of sulphur into long-chain polysulphides and the lower discharge plateau represents the conversion of short-chain polysulphides (Li 2 S 2 /Li 2 S), which are reminiscent in the charge plateaus as well [8] . The discharge capacity values of the cell at the first, second and 50th cycle at 1C rate are identical, except for the length ratio between the upper ( Q up ) and lower ( Q low ) plateaus. A much higher Q low / Q up ratio of 2.10 can be observed in the cell after 50 cycles compared with that after the first cycle ( Q low / Q up =1.06). As the representative microporous carbon–sulphur composite cathodes exhibit only the lower discharge plateau during cycling [16] , [18] , the stretching Q low corresponds to the capacity contribution from the micropore-trapped active material. In addition, it appears that the active material needs to take a few cycles to reach a steady state in the cathode region to offer stable electrochemical performance because of the solubility of the intermediate lithium polysulphides in the electrolyte [14] . The inactive core of sulphur cannot be reutilized until it becomes exposed to the electrolyte after the initial cycles at high C rates [25] , which is evident in the second cycle where the discharge capacity is even higher than the first charge capacity ( Fig. 3c ). Figure 3: Electrochemical measurements of Li–S batteries. ( a ) Electrochemical impedance spectroscopy plots of Li–S cells with and without MCP, ( b ) cyclic voltammogram scans, ( c ) discharge/charge profiles at various cycles, ( d ) rate capability up to 3C and ( e ) cycle life and Coulombic efficiency of the cell with MCP at 1C and 2C for long cycles. Full size image The rate capability of the cell with the MCP is shown in Fig. 3d . The C rates specified in this study are based on the mass and theoretical capacity of sulphur (1C=1,675 mA g −1 ). The first discharge capacity is as high as 1,367 mA h g −1 , demonstrating the assistance of the effective carbon interlayer in enhancing the conductivity and active material utilization. The cell with the MCP could be cycled up to 3C, whereas maintaining a capacity above 846 mA h g −1 for 70 cycles. As exhibited in Fig. 3e , the cyclability at 1C rate retains over 1,000 mA h g −1 after 100 cycles, converting to a retention rate of 85% with an average Coulombic efficiency of 97.6%. The charge efficiency of the first 2 cycles is higher than 100% due to the re-utilization of the sulphur core in the cathode as the cell is cycled. The re-utilization of the inactive core of the active material is generally found in the Li–S system, especially at high C rates during the initial cycles. At a higher rate of 2C for long cycles, the cell with the MCP exhibits 846 mA h g −1 with an average Coulombic efficiency of >98% after 150 cycles; it also shows a more considerable capacity increase during the first 40 cycles compared with the cell at a 1C rate. We also tested another bimodal micro-/mesoporous carbon paper (micropores ~1.5 nm; mesopores ~6 nm) as an interlayer in Li–S cells; however, the battery performance was not as good as the one with the microporous carbon interlayer under the same conditions. Active sulphur in the battery first transforms to long-chain Li 2 S 8 , which consists of two Li–S bonds and seven S–S bonds. Both bond types have a bond length of about 2 Å [26] , [27] , so the longest chain length estimated among the species of polysulphides (Li 2 S 8 ) is around 2 nm. Therefore, much larger pores like mesopores may not trap the migrating polysulphides efficiently during cycling because of the size effect. In contrast, microporous/small-mesoporous materials possess the advantage to absorb polysulphide intermediates due to the similar dimensions of the pores and polysulphide ions, thereby enhancing the cycling reversibility of Li–S batteries. In summary, a microporous carbon interlayer has been developed to substantially improve the cycle performance of the Li–S batteries. The flexible carbon paper provides fine contact with the cathode surface, offering electron pathways through the insulating S/Li 2 S and accommodating the migrating polysulphide intermediates. This bifunctional carbon interlayer with micropores/small-mesopores operates not only as an “upper current collector” to enhance the active material utilization but also as a “polysulphide stockroom” to retain the cyclability. Moreover, the cells involve only a novel cell configuration by inserting an interlayer without requiring the formation of sulphur–carbon or sulphur–polymer composites, leading to facile and low-cost manufacturing. This strategy can be extended with other potential lightweight conductive/porous interlayers, offering further improvement in Li–S batteries. Synthesis and characterization The MCP samples were prepared by mixing conductive carbon black with high surface area (Black Pearls 2000, CABOT) and polytetrafluoroethylene binder at a 3:2 mass ratio, with a small amount of isopropyl alcohol in a mortar, followed by roll-pressing and cutting into circular films. The microstructure of the samples was examined with a FEI Quanta 650 SEM and a JEOL JEM-2010F transmission electron microscope. Brunauer−Emmett−Teller surface area measurements were carried out with a volumetric sorption analyser (NOVA 2000, Quantachrome) using physical adsorption/desorption of nitrogen gas at the liquid-nitrogen temperature. Pore size distributions were calculated according to the Barrett–Joyner–Halenda method. Micropore surface area and volume were estimated by the t -plot method. Cell assembly Sulphur cathode slurry was fabricated by mixing 70 wt% of precipitated sulphur, 20 wt% of carbon black (Super P) and 10 wt% of polyvinylidene fluoride (Kureha) binder in an N -methylpyrrolidinone (Sigma-Aldrich) solution overnight. The slurry was tape-casted onto an aluminium foil and dried in an air oven for 24 h at 50 °C, followed by roll-pressing and cutting into circular electrodes. The cathode disks and MCP interlayers were dried in a vacuum oven for an hour at 50 °C before assembling the cell. The electrolyte was prepared by adding 1.85 M LiCF 3 SO 3 (Acros Organics) and 0.1 M LiNO 3 (Acros Organics) salts into a mixture of 1,2-dimethoxyethane (Acros Organics) and 1,3-dioxolane (Acros Organics) at a 1:1 volume ratio. CR2032 coin cells were assembled with the sulphur cathodes, prepared electrolyte, MCP interlayers, polypropylene separators (Celgard) and lithium foils (Aldrich). Electrochemistry Electrochemical impedance spectroscopy data were obtained with a Solartron Impedance Analyser (SI 1,260+SI 1,287) from 1 to 100 mHz with an AC voltage amplitude of 5 mV at the open-circuit voltage of the cells with the Li metal foil as both auxiliary and reference electrodes. Discharge/charge profiles and cycle data were collected with a programmable battery cycler (Arbin Instruments). The cyclic voltammogram plots were collected with a VoltaLab PGZ 402 Potentiostat at a scan rate of 0.2 mV s −1 in the voltage window of 2.8–1.5 V. Morphological characterization and elemental mapping of the MCP samples before and after cycling were carried out with a Hitachi S-5500 SEM equipped with an energy-dispersive spectrometer. How to cite this article: Su, Y.-S. & Manthiram, A. Lithium–sulphur batteries with a microporous carbon paper as a bifunctional interlayer. Nat. Commun. 3:1166 doi: 10.1038/ncomms2163 (2012).